JAK2V617Fmutation drives vascular resident macrophages toward a pathogenic phenotype and promotes dissecting aortic aneurysm JAK2V617F mutation is associated with an increased risk for athero-thrombotic cardiovascular disease, but its role in aortic disease development and complications remains unknown. In a cohort of patients with myeloproliferative neoplasm, JAK2V617F mutation was identified as an independent risk factor for dilation of both the ascending and descending thoracic aorta. Using single-cell RNA-seq, complementary genetically-modified mouse models, as well as pharmacological approaches, we found that JAK2V617F mutation was associated with a pathogenic pro-inflammatory phenotype of perivascular tissue-resident macrophages, which promoted deleterious aortic wall remodeling at early stages, and dissecting aneurysm through the recruitment of circulating monocytes at later stages. Finally, genetic manipulation of tissue-resident macrophages, or treatment with a Jak2 inhibitor, ruxolitinib, mitigated aortic wall inflammation and reduced aortic dilation and rupture. Overall, JAK2V617F mutation drives vascular resident macrophages toward a pathogenic phenotype and promotes dissecting aortic aneurysm. Aortic aneurysm (AA) is a frequent vascular disease affecting approximately 5% of elderly men in Western countries [1] whose incidence is still increasing despite better control of risk factors like smoking and blood pressure. Surgery and endovascular procedure are the only treatments for individuals with aortic aneurysm to limit the risk of aortic rupture and dissection, but the interventions are costly and associated with high morbidity and mortality [2] . Currently, no drug treatments have been approved for use in aortic aneurysm, which underlines the need for a better understanding of mechanisms underlying the disease in order to implement novel management procedures and therapeutic strategies. The mechanisms of aortic aneurysm formation are complex, including elastin degradation, collagen remodeling, smooth muscle cell apoptosis and local activation of immune cells such as macrophages [3] . Several experimental studies have suggested that during the first stages of AA formation, circulating monocytes interact with activated endothelial cells (ECs) and are recruited into the aortic wall, Ly6C high monocytes dominating the acute phase of injury while non-classical Ly6C low monocytes being prevalent thereafter [4] . Recruitment into the vascular wall depends, at least in part, on GM-CSF [5] , chemokines/chemokine receptors [6] , and adhesion molecules. Monocytes locally differentiate into macrophages and, after activation, promote aneurysm formation and complications (dissection and/or rupture) through the release of inflammatory cytokines (including TNF-α, IL-1β) and matrix metalloproteinases (MMPs). Another subset of macrophages, tissue-resident macrophages, which originate from the yolk sac and fetal liver during development [7] , [8] , has been recently identified as essential for the maintenance of arterial wall homeostasis through the regulation of smooth muscle cell activity and collagen production [9] . Tissue-resident macrophages express the lymphatic vessel endothelial hyaluronan receptor-1 (LYVE-1), but their role in aortic aneurysm formation and progression remains unknown. JAK2V617F is a gain-of-function mutation responsible for enhanced hypersensitivity to growth factors and cytokines [10] . JAK2V617F mutation promotes the proliferation, the survival and the maturation of hematopoietic progenitors leading to myeloproliferative neoplasms such as polycythemia vera, essential thrombocythemia, and primary myelofibrosis [10] , [11] . The presence of JAK2V617F mutation is associated with an increased risk of cardiovascular diseases [12] . Experimental studies have shown that JAK2V617F mutation in bone marrow cells, mimicking human myeloproliferative neoplasms, accelerates atherosclerosis in hypercholesterolemic mice due to impaired red blood cell efferocytosis and inflammasome activation [13] , and aggravates post-ischemic cardiac remodeling [14] . However, the role of JAK2V617F mutation in aortic aneurysm development and complications has never been investigated. Here, we showed that JAK2V617F mutation is associated with aortic dilation in patients. Moreover, using several complementary genetic and pharmacological approaches in murine models, we found that JAK2V617F mutation drives adventitial tissue-resident macrophages toward a pathogenic inflammatory phenotype causing aortic aneurysm and dissection. Global JAK2V617F mutation promotes aortopathy in humans, and aortic aneurysm and dissection in mice Several epidemiological studies have shown that JAK2V617F gain-of-function mutation is associated with increased risk for athero-thrombotic cardiovascular disease, but to our knowledge nothing has been reported regarding the possible association between this mutation and aortic disease. To address this issue, we first screened JAK2V617F + patients recruited at Saint-Antoine Hospital ( N = 382, Paris, France), and identified those who had a recent Body CT-scan ( N = 157/382). Mean diameter was measured in different segments of the aorta (ascending, descending thoracic and abdominal) and compared to age- and gender-matched controls by a blinded independent reader (Supplementary Fig. 1 ). 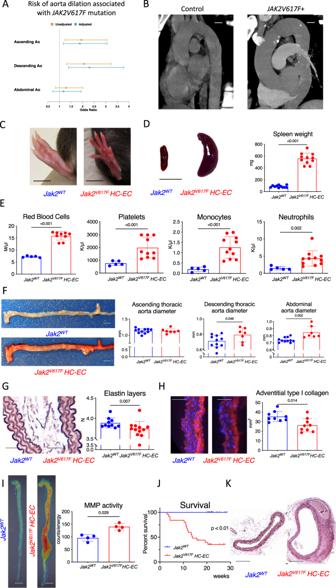Fig. 1: JAK2V167F mutation leads to aortopathy in both human and mice. AAdjusted risk factor for aorta dilation in a cohort ofJAK2V167F+ patients (n= 157) and age-gender-matched controls (N= 157), scale bar 2 cm.BCT-scan 3D-reconstruction ofJAK2V167F+ patient (right) and control (left) showing ascending and descending thoracic aorta.CPaw pictures of 7-week-oldJak2WTcontroland Jak2V617FHC-ECmice showing palmar erythema in mutant mice, scale bar 1 cm.DQuantitative analysis and representative photomicrographs of spleen size in 7-week-old controlJak2WT(N=11) and Jak2V617FHC-ECmice (N= 11) (scale bar 1 cm).Ered blood cell, platelet, and myeloid cell count of 7-week-old controlJak2WT(N=5) and Jak2V617FHC-ECmice (N= 9).FRepresentative photomicrographs and quantitative analysis of the mean aortic diameter in 7-week-old controlJak2WT(N=11) and Jak2V617FHC-ECmice (N= 7) in the thoracic (ascending and descending) and the abdominal aorta (scale bar 1 mm).GQuantification of the number of elastin layers in the aortic wall by orcein staining in 7-week-old animals (N= 10–12/group), scale bar 50 μm.HQuantification of the collagen content (Cola1 immunostaining) in the aortic wall in 7-week-old animals (N = 9/group), scale bar 50 μm.IFluorescent Molecular Tomography quantification of matrix metalloproteinase (MMP-2, −3, −9 and −13) activity in aorta of 10-week-old animals (N= 4/group), scale bar 1 mm.JSurvival curve of controlJak2WT(N= 15)and Jak2V617FHC-ECmice (N= 25).KRepresentative photomicrographs of descending thoracic aorta after Orcein staining showing dissecting aortic aneurysm inJak2V617FHC-ECmouse (representative of 10 aortas/group), scale bar 100 µm. Data are presented as mean values ± SD. [Two-tailed Mann-Whitney test, *P< 0.05, **P< 0.01, ***P< 0.001]. Difference in survival was evaluated using log-rank test.CTcomputed tomography,HC-EChematopoietic cells-endothelial cells,MMPmatrix metalloprotease. Source data are provided as a Source Data file. General characteristics of the cohort are detailed in Supplementary Table 1 . Interestingly, after multiple adjustment on age, gender, hypertension, diabetes and smocking, we found that the JAK2V617F mutation was associated with significant dilation of both ascending and descending thoracic aorta, but not abdominal aorta (Fig. 1A, B ). Fig. 1: JAK2V167F mutation leads to aortopathy in both human and mice. A Adjusted risk factor for aorta dilation in a cohort of JAK2V167F + patients ( n = 157) and age-gender-matched controls ( N = 157), scale bar 2 cm. B CT-scan 3D-reconstruction of JAK2V167F + patient (right) and control (left) showing ascending and descending thoracic aorta. C Paw pictures of 7-week-old Jak2 WT control and Jak2 V617F HC-EC mice showing palmar erythema in mutant mice, scale bar 1 cm. D Quantitative analysis and representative photomicrographs of spleen size in 7-week-old control Jak2 WT (N = 11) and Jak2 V617F HC-EC mice ( N = 11) (scale bar 1 cm). E red blood cell, platelet, and myeloid cell count of 7-week-old control Jak2 WT (N = 5) and Jak2 V617F HC-EC mice ( N = 9). F Representative photomicrographs and quantitative analysis of the mean aortic diameter in 7-week-old control Jak2 WT (N = 11) and Jak2 V617F HC-EC mice ( N = 7) in the thoracic (ascending and descending) and the abdominal aorta (scale bar 1 mm). G Quantification of the number of elastin layers in the aortic wall by orcein staining in 7-week-old animals ( N = 10–12/group), scale bar 50 μm. H Quantification of the collagen content (Cola1 immunostaining) in the aortic wall in 7-week-old animals (N = 9/group), scale bar 50 μm. I Fluorescent Molecular Tomography quantification of matrix metalloproteinase (MMP-2, −3, −9 and −13) activity in aorta of 10-week-old animals ( N = 4/group), scale bar 1 mm. J Survival curve of control Jak2 WT ( N = 15) and Jak2 V617F HC-EC mice ( N = 25). K Representative photomicrographs of descending thoracic aorta after Orcein staining showing dissecting aortic aneurysm in Jak2 V617F HC-EC mouse (representative of 10 aortas/group), scale bar 100 µm. Data are presented as mean values ± SD. [Two-tailed Mann-Whitney test, * P < 0.05, ** P < 0.01, *** P < 0.001]. Difference in survival was evaluated using log-rank test. CT computed tomography, HC-EC hematopoietic cells-endothelial cells, MMP matrix metalloprotease. Source data are provided as a Source Data file. Full size image In order to understand the cellular and molecular mechanisms responsible for aortopathy in JAK2V617F + patients, we used genetically-modified mouse models. First, we studied Jak2V617F WT/Flex VE-Cadherin -Cre+/- mice, herein referred to as Jak2 V617F HC-EC mice, in which Cre-mediated recombination occurs in ECs and hematopoietic cells (HCs) due to the expression of VE-cadherin during early embryonic life in a precursor of both ECs and HCs [15] , [16] (Supplementary Fig. 2A ). Jak2 V617F HC-EC mice developed myeloproliferative neoplasm, as attested by palmar erythema (Fig. 1C ), splenomegaly (87 ± 27 vs 560 ± 81 mg; P < 0.0001) (Fig. 1D ), and higher red blood cell, platelet and leukocyte counts than littermate controls (Fig. 1E & Supplementary Fig. 2B ). At 7 weeks, we performed histological analysis and we found aortic dilation in Jak2 V617F HC-EC mice affecting descending thoracic (0.71 ± 0.07 vs 0.80 ± 0.08 mm, P < 0.05) and abdominal (0.74 ± 0.03 vs 0.85 ± 0.08 mm, P < 0.01) aortic regions (Fig. 1F ). Notably, both systolic and diastolic blood pressure were significantly lower in Jak2 V617F HC-EC mice than in littermate controls, which rules out the possibility that aortic dilation resulted from hypertension (Supplementary Fig. 2C ). At 7 weeks of age, hematopoietic and endothelial JAK2V617F gain-of-function mutation was associated with enhanced elastin degradation, as assessed by the significantly lower number of elastin layers in the abdominal aorta of Jak2 V617F HC-EC mice compared with the aorta of control Jak2 WT HC-EC mice (3.90 ± 0.12 vs 3.70 ± 0.17 layers, P < 0.05) (Fig. 1G ), and reduced content in collagen type 1a (Fig. 1H & Supplementary Fig. 2D ), but no difference in α-SMA + smooth muscle cell content (Supplementary Fig. 2E ). The decrease in extracellular matrix protein content in Jak2 V617F HC-EC mice was accompanied with an increase in global MMP activity in the aortic wall, quantified using ex vivo fluorescence molecular tomography imaging (Fig. 1I ) and qPCR (Supplementary Fig. 2F ). Interestingly, we observed specifically in Jak2 V617F HC-EC mice spontaneous early death (Fig. 1J & Supplementary Fig. 2G ), reaching 70% at 20 weeks of age; which was due to aortic dissecting aneurysm (Fig. 1K ) and thoracic and/or abdominal hemorrhage. Polyglobulia correction using phenylhydrazine [17] in Jak2 V617F HC-EC mice did not impact either on aorta dilation or rupture incidence (Supplementary Fig. 3 ). JAK2V617F mutation specifically expressed in vascular cells did not induce dissecting aortopathy To assess the implication of JAK2V617F mutation in vascular cells, we used 2 complementary approaches. First, we generated chimeric mice expressing JAK2V617F mutation only in non-hematopoietic cells by transplanting C57BL/6 bone marrow (BM) cells into lethally irradiated Jak2 V617F HC-EC mice and C57BL/6 controls (Supplementary Fig. 4A ) [16] . BM cell transplantation after irradiation allows hematopoietic reconstitution, including perivascular LYVE-1 + tissue-resident macrophages (Supplementary Fig. 5 ). JAK2V617F mutation only in vascular cells did not induce myeloproliferative neoplasm (Supplementary Fig. 4B ) and did not induce elastin degradation (Supplementary Fig. 4D ) or aortic dilation (Supplementary Fig. 4C ). Moreover, no death was recorded during the 3-month follow-up in the 2 groups of chimeric mice (Supplementary Fig. 4E ). In order to investigate the role of JAK2V617F mutation specifically in endothelial cells in the onset of spontaneous dissecting aortopathy, we next generated Jak2V617F WT/Flex VE-cadherin-Cre-ERT2 (herein referred to as Jak2 V617F EC ) mice. We crossed Jak2V617F WT/Flex mice with inducible VE-cadherin-Cre-ERT2 mice expressing the Cre recombinase after tamoxifen injection only in endothelial cells (Supplementary Fig. 6A ). The absence of hematopoietic recombination in this model, as well as adequate endothelial recombination has been previously validated [16] , [18] . As expected, mice did not develop myeloproliferative neoplasm (Supplementary Fig. 6B ). Aortic wall structure was preserved in mice expressing JAK2V617F mutation in endothelial cells (Supplementary Fig. 6D ). In Jak2 V617F EC mice, we observed neither aortic dilation (Supplementary Fig. 6C ) nor premature death (Supplementary Fig. 6E ). Altogether, these experiments indicate that JAK2V617F mutation in vascular cells was not responsible for dissecting aortopathy. JAK2V617F mutation specifically expressed in myeloid cells induces dissecting aortopathy To assess the implication of JAK2V617F mutation in hematopoietic cells, we generated chimeric mice expressing JAK2V617F mutation only in hematopoietic cells by transplanting BM cells from Jak2 V617F HC-EC mice into lethally irradiated C57BL/6 mice. Irradiated C57BL/6 mice transplanted with C57BL/6 BM cells were used as controls (Fig. 2A ). Hematopoietic expression of JAK2V617F induced a myeloproliferative neoplasm (Fig. 2B ), elastin degradation (Fig. 2C ) and spontaneous aortic dilation at 1 (Supplementary Fig. 7A ) and 3 months (Fig. 2D ) after BMT. In addition, irradiated C57BL/6 mice were transplanted with 100% Jak2 WT BM cells or a mixture of 80% Jak2 WT /20% Jak2 V617F HC-EC BM cells. One month after BMT, we observed aorta dilation in chimeric mice receiving 20% Jak2 V617F BM cells, despite no major changes in blood cell subsets (Supplementary Fig. 7B, C ). Fig. 2: JAK2V167F mutation in hematopoietic cells promoted dissecting aortopathy. A Experimental protocol of WT or Jak2 V617F HC-EC bone marrow cell transplantation in lethally irradiated C57BL/6 mice (7/Group). B Red blood cell, white blood cell and platelet count of 20-week-old chimeric mice ( N = 7/group). C Quantification of the number of elastin layers in the aortic wall by Orcein staining at sacrifice ( N = 7/group), scale bar 50 μm. D Representative photomicrographs and quantitative analysis of the mean aortic diameter in WT or Jak2 V617F HC-EC chimeric mice ( N = 7/group) in the thoracic (ascending and descending) and the abdominal aorta, scale bar 0.5 mm. E Red blood cell, white blood cell and platelet count of 7-week-old Jak2 WT and Jak2 V617F Myel mice ( N = 7/group). F Quantification of the collagen content (Cola1 immunostaining) in the aortic wall in 7-week-old Jak2 WT ( N = 6) and Jak2 V617F Myel animals ( N = 8), scale bar 50 μm. G Quantification of Cola1 and Cola3 mRNA expression in aorta of 7-week-old Jak2 WT ( N = 7) and Jak2 V617F Myel mice ( N = 8). H Fluorescent Molecular Tomography quantification of matrix metalloproteinase (MMP-2, −3, −9, and −13) activity in aorta of 9-week old Jak2 WT and Jak2 V617F Myel mice ( N = 4/group), scale bar 1 mm. I, quantification of Mmp2, Mmp3, Mmp9, Mmp12, Mmp13 mRNA expression in aorta of 7-week-old Jak2 WT ( N = 5) and Jak2 V617F Myel mice ( N = 7). J Representative photomicrographs and quantitative analysis of the mean aortic diameter in 7-week-old Jak2 WT ( N = 7) and Jak2 V617F Myel ( N = 8 ) mice in the thoracic (ascending and descending) and the abdominal aorta, scale bar 1 mm. K Survival curve of Jak2 WT ( N = 11) and Jak2 V617F Myel mice ( N = 14). Data are presented as mean values ± SD. [Two-tailed Mann-Whitney test, * P < 0.05, ** P < 0.01, *** P < 0.001]. Difference in survival was evaluated using log-rank test. HC-EC, hematopoietic cells-endothelial cells; MMP, matrix metalloprotease. Source data are provided as a Source Data file. Full size image Next, to evaluate the implication of JAK2V617F in myeloid cells, we crossed Jak2V617F WT/Flex mice with LysMCre ± mice expressing the Cre recombinase under Lysozyme M promoter, mainly expressed in myeloid cells (Supplementary Fig. 7D ). Jak2V617F WT/Flex LysMCre +/− , referred to as Jak2 V617F Myel , developed myeloproliferative neoplasm, as attested by palmar erythema (Supplementary Fig. 7E ), splenomegaly (Supplementary Fig. 7F ), and higher number of circulating red blood cells, neutrophils and monocytes compared to littermate controls. However, platelet count was not different between groups (Fig. 2E ). Histological analysis of aorta from 7-week-old Jak2 V617F Myel mice phenocopied the vascular phenotype of Jak2 V617F HC-EC mice. Indeed, JAK2V617F gain-of-function mutation under LysM promoter led to elastin degradation, as assessed by the significantly lower number of elastin layers in the abdominal aorta of Jak2 V617F Myel mice compared with the aorta of control Jak2 WT Myel mice (4.5 ± 0.24 vs 4.2 ± 0.09 layers, P < 0.05) (Supplementary Fig. 7G ), which was associated with a reduction in collagen type 1a content (Fig. 2F, G ) but no difference in α-SMA + smooth muscle cells content (Supplementary Fig. 7H ). Global MMP activity in the aortic wall of Jak2 V617F Myel mice was significantly increased (Fig. 2H, I ). At 7 weeks of age, we observed dilation in ascending thoracic (0.90 ± 0.06 vs 1.12 ± 0.05 mm, P < 0.05), descending thoracic (0.66 ± 0.12 vs 0.86 ± 0.10 mm, P < 0.05) and abdominal (0.72 ± 0.12 vs 0.89 ± 0.11 mm, P < 0.05) aorta in Jak2 V617F Myel mice, compared to Jak2 WT Myel mice (Fig. 2J ). Finally, we observed that all Jak2 V617F Myel mice (100%) spontaneously died before 15 weeks of age. Autopsy was systematically performed and confirmed that deaths were due to dissecting aortic aneurysm, mainly associated with thoracic and/or abdominal hemorrhage (Fig. 2K ). Taken together, these findings demonstrate that the presence of the JAK2V617F mutation in myeloid cells was responsible for the development of dissecting aortic aneurysm. In order to understand the mechanisms underlying the lethal JAK2V617F -dependent aortic disease, we performed RNA sequencing of the aorta of 7-week-old Jak2 V617F HC-EC and control Jak2 WT mice. The whole transcriptomic profile of the aorta was markedly altered by JAK2V617F global mutation, with upregulation of the expression of 137 genes and downregulation of the expression of 70 genes (Fig. 3A ). Gene Ontology analysis showed that inflammatory pathways were upregulated in Jak2 V617F HC-EC aorta, including those associated with myeloid cell differentiation, homeostasis and development (Fig. 3B ). Based on this finding, we investigated the consequences of JAK2V617F mutation on the local inflammatory response. First, we analyzed the immune cell composition in aorta of 7-week-old Jak2 V617F HC-EC mice and controls by flow cytometry, after enzymatic digestion. We did not find any significant differences in monocyte and neutrophil counts (Fig. 3C & Supplementary Fig. 8A ), but we observed a 3-fold increase in CD45 + CD11b + Ly6G - F4/80 high CD68 high macrophages in the aorta from Jak2 V617F HC-EC mice ( P < 0.05) (Fig. 3D ). This result was confirmed by immunostaining in Jak2 V617F HC-EC (Fig. 3E ) and Jak2 V617F Myel mice (Supplementary Fig. 8B ). The significant increase in Il1β, Il6 and Tnfα mRNA expression in aorta of Jak2 V617F HC-EC mice supports a vascular pro-inflammatory immune response in mutant mice (Fig. 3F ). Notably, most of vascular CD68 + macrophages in mutant mice with aortic dilation expressed LYVE-1 (Fig. 3G ) and a significant number expressed Ki-67, a proliferation marker (Supplementary Fig. 8 C). However, at more advanced stage, most of CD68 + macrophages in Jak2 V617F HC-EC mice with severe aortic aneurysm did not colocalize with LYVE-1 + staining (Fig. 3G ). All these observations suggest that macrophage accumulation in mutant mice at early stages unlikely resulted from the differentiation of infiltrating blood monocytes, but most likely from an expansion of tissue-resident macrophages. Transcriptomic analysis confirmed that genes related to the phenotype of tissue-resident macrophages ( F13a1, Lyve1, Pf4, and Gas6 ) [19] were enriched in the aorta of Jak2 V617F HC-EC mice (Fig. 3H ). Fig. 3: JAK2V167F mutation induces pro-inflammatory signature in the aortic wall. A Difference in gene expression in the aorta of 7-week-old Jak2 WT ( N = 4) and Jak2 V617F HC-EC mice ( N = 3). B Top Gene Ontology terms mostly enriched among genes upregulated in the aorta of Jak2 V617F HC-EC mice when compared to Jak2 WT mice . C Flow cytometry quantification of CD45 + CD11c low CMHII low CD11b + Ly6G-F4/80 low CD64 low Ly6C + monocytes and CD45 + CD11c low CMHII low CD11b + Ly6G+ neutrophils in the aorta of 7-week-old Jak2 WT ( N = 10) and Jak2 V617F HC-EC animals ( N = 8). D Flow quantification and representative dot plot of CD45 + CD11c low CMHII low CD11b + Ly6G-F4/80 high CD64 high macrophage count in the aorta of 7-week-old Jak2 WT ( N = 10) and Jak2 V617F HC-EC animals ( N = 8). E Quantification and representative photomicrographs of CD68 positive macrophages in the aorta of 7-week-old mice ( N = 11 in control group and N = 8 in Jak2 V617F HC-EC group), scale bar 50 µm. F Quantification of Il6, Tnfα, Il1β, and Il10 mRNA expression by RT-qPCR in the aorta of 7-week-old Jak2 WT ( N = 8) and Jak2 V617F HC-EC animals ( N = 9). G Immunofluorescence staining in the aortic wall of Jak2 WT and Jak2 V617F HC-EC mice, DAPI (Blue), CD68 (Red), LYVE-1 (Green), scale bar 50 μm. resident macrophages were defined as CD68 + LYVE-1+ cells ( N = 5/group). H GSEA for genes related to a gene set signature for tissue resident macrophage [19] in the aorta of 7-week-old Jak2 WT and Jak2 V617F HC-EC animals ( N = 4/group). Data are presented as mean values ± SD. [Two-tailed Mann-Whitney test, * P < 0.05, ** P < 0.01, *** P < 0.001]. HC-EC, hematopoietic cells-endothelial cells; Il , interleukin; Tnf , tumor necrosis factor; GSEA, gene set enrichment analysis. Source data are provided as a Source Data file. Full size image Jak2V617F Myel aortas harbor pro-inflammatory Lyve1 + resident macrophages To better characterize aortic macrophage populations in Jak2 V617F Myel mice, we performed cellular indexing of transcriptomes and epitopes by sequencing (CITE-seq) [20] of total CD45 + cells from Jak2 WT ( n = 5) and Jak2 V617F Myel ( n = 5) aortas (Fig. 4A ). At sacrifice, among Jak2 V617F Myel mice, macroscopically observable aortopathy was seen in all mice, 2 mice displayed aortic aneurysm and 3 mice exhibited aortic dilation. Based on the expression of canonical cell surface markers and lineage-specific transcripts, immune cell subsets were identified and annotated (Fig. 4B , Supplementary Fig. 9A, B ). Cells corresponding to monocytes/macrophages were extracted and reclustered separately to better resolve discrete subpopulations (Fig. 4A–C ). We recovered several populations of LYVE-1 + tissue-resident macrophages ( Lyve1, Mrc1 ; surface CD163, TIMD4, CD169, Fig. 4D ) and recruited monocytes/macrophages ( Ccr2 ; surface CD14, Fig. 4D ). Differential gene expression analysis revealed three distinct populations of LYVE-1 + tissue-resident macrophages: Res-MGL1 hi (cluster A, enriched in Clec10a encoding MGL1), Res- Txnip hi (cluster B: Txnip, Trf, Stab1 ) and Res-S100 hi (cluster C enriched in S100-protein encoding genes such as S100a4 , S100a6 or S100a10 ) (Fig. 4C–E ). Ccr2 + inflammatory macrophages (cluster D) were enriched for e.g. Spp 1, Tnip3 or Il1b (Fig. 4C–E ). Populations of type I IFN response macrophages (IFNIC, cluster E: [21] Isg15, Ifit ), monocytes (cluster F: Plac8, Ly6c2, Chil3 , surface Ly6C), and macrophages with high expression of early immediate-early genes [22] (cluster G, IEG + : Egr1, Zfp36 ) were also detected (Fig. 4C–E ). Fig. 4: Jak2 V617F Myel aortas harbor pro-inflammatory Lyve1 + tissue resident macrophages. A Experimental design, B UMAP visualization of scRNA-seq profiles of CD45 + cells extracted from Jak2 WT and Jak2 V617F Myel aortas. C Single-cells annotated as macrophages on the UMAP displayed in B were in silico extracted, reanalyzed with dimensional reduction (UMAP) and clustered identifying 7 major populations (Annotated A to G). D Expression intensity of transcripts (top) and cell surface markers (bottom) characteristic of tissue resident macrophages (Lyve1, Mrc1, TIMD4, CD169) and recruited monocytes/macrophages (Ccr2, CD14) projected on the macrophage UMAP plot. E Expression of selected marker transcripts in the 7 macrophage populations. F Macrophage UMAP plot split according to experimental condition (color code as in B ). G Proportions of macrophage populations among total aortic macrophages. H Proportions of tissue resident macrophage subsets among total aortic tissue resident macrophages. I Normalized expression of the indicated transcripts in tissue resident macrophage subpopulations. J Average expression of the indicated cell surface markers (measured by CITE-seq) in tissue resident macrophage subpopulations. UMAP, Uniform Manifold Approximation and Projection for Dimension Reduction, sc single cell, CITE-seq Cellular Indexing of Transcriptomes and Epitopes by Sequencing. Full size image Distribution of macrophage subpopulations was dependent on genotype and disease severity. Pro-inflammatory Ccr2 + macrophages were particularly abundant in aortic aneurysm (59.6% of macrophages), while they were relatively rare in Jak2 WT and Jak2 V617F Myel with limited aortic dilation (Fig. 4F, G ), consistent with our observation of infiltration of Lyve1 - macrophages in the media of mutant mice with severe aortic aneurysm (Fig. 3G ). The distribution of the different subsets of tissue-resident macrophages differed according to the genotype. Res-MGL1 hi were preferentially found in Jak2 V617F Myel aortas regardless of aortic disease severity (61.4% and 56.0% of tissue-resident macrophage in Jak2 V617F Myel aortas with aortic aneurysm and dilation, respectively), and Res- Txnip hi were more abundant in Jak2 WT aortas (60.2% of tissue-resident macrophages), whereas Res-S100 hi macrophages were evenly distributed across genotypes (Fig. 4G ). Moreover, all resident macrophage populations shared expression of markers previously reported as associated with aortic resident macrophages ( Lyve1, Folr2, Cbr2, F13a1, Gas6 ) (Fig. 4D and Supplementary Fig. 9 ) [7] , [19] , [23] , but Res-MGL1 hi macrophages, particularly abundant in Jak2 V617F Myel aortas, showed higher expression of pro-inflammatory transcripts ( Nlrp3, Tnf, Tnfsf9, Ccl2, Cxcl1, Cxcl2, Cxcl10 ) (Fig. 4I ). Interestingly, Lyve1 expression was significantly increased in Res-MGL1 hi compared to Res- Txnip hi macrophages, in agreement with our finding of higher expression levels of Lyve1 observed in bulk tissue transcriptome analysis of Jak2 V617F HC-EC aortas (Fig. 3H ). Differential expression of cell surface markers measured by CITE-seq indicated that besides MGL1, Res-MGL1 hi macrophages exhibited higher surface levels of pro-inflammatory proteins such as CD95 (Fas), CD178 (Fas-Ligand), CD40 or JAML (Fig. 4J ). All these data confirmed a pro-inflammatory signature in the aorta of Jak2 V617F Myel mice but pathways related to angiogenesis and lymphoangiogenesis were not impaired in mutant aortas (Supplementary Fig. 10A, B ). Altogether, these results indicate that JAK2V617F mutation in myeloid cells not only increased the number of aortic resident Lyve-1 + macrophages, but also polarized them towards a pro-inflammatory pathogenic phenotype. The JAK2V617F mutation in vascular tissue-resident macrophages induces dissecting aortic aneurysm We then sought to generate a genetic model in which the JAK2V617F mutation would be preferentially induced in the tissue-resident macrophages. Our selection of an adequate Cre-driver was guided by data obtained from scRNA-seq analysis. Previous scRNA-seq studies have identified Platelet factor 4 ( Pf4 ), highly expressed in megakaryocytes, as a marker of aortic resident macrophages [19] , [24] , which we confirmed using an integrated dataset combining several independent single-cell studies of healthy and diseased mouse aortas [25] (Fig. 5A ). Likewise, in our newly generated data, Pf4 was highly expressed in LYVE-1 + resident macrophage subsets, but at much lower levels in CCR2 + inflammatory macrophages and monocytes (Fig. 5B ). In scRNA-seq data from mouse blood CD11b + cells [26] , Pf4 expression was absent from monocytes, but readily detected in contaminating platelets (Supplementary Fig. 11A ). In line with our scRNA-seq analysis, previous studies using fluorescent reporter have demonstrated efficient Pf4 -Cre-induced recombination in CD206 + LYVE-1 + perivascular macrophages [24] , but limited recombination in circulating monocytes [27] . Based on these findings, we crossed Jak2V617F WT/Flex mice with Pf4 Cre+/- mice expressing the Cre recombinase under Pf4 promoter, to generate transgenic mice with a preferential recombination of JAK2V617F mutation in tissue-resident macrophages (Fig. 5C ). Jak2V617F Flex Pf4 Cre+/- mice, referred to as Jak2 V617F Pf4 , developed aortic dilation and aneurysm before red blood cell and white blood cell increased in the blood. Indeed, at 7 weeks of age, red blood cell and white blood cell counts in the blood were not different between Jak2 V617F Pf4 and Jak2 WT controls (Fig. 5D ), but the aorta was significantly dilated in Jak2 V617F Pf4 mice (Fig. 5E, F ), associated with reduced peri-adventitial collagen 1a content (Fig. 5G, H ), increased MMP signature (Fig. 5I ) and marked accumulation of LYVE-1 + macrophages (Fig. 5J ). The significant increase in Il6 and Tnfα mRNA expression in aorta of Jak2 V617F Pf4 mice supports a vascular pro-inflammatory immune response in mutant mice (Fig. 5K ). During the follow-up, 89% (34/38) of Jak2 V617F Pf4 mice spontaneously died of dissecting aortic aneurysm, whereas only one death was observed in the control group (1/28, 4%) ( P < 0.0001) (Fig. 5L ). Fig. 5: JAK2 mutation in vascular tissue resident macrophage cells promotes dissecting aortopathy. A Left, cells corresponding to monocytes/macrophages/dendritic cells were extracted from murine healthy and atherosclerotic plaques and separately reanalyzed with dimensional reduction (UMAP) [25] . Right, expression of Pf4 transcript projected on the vascular monocytes/macrophages/dendritic cells UMAP plot. B Left, cells corresponding to macrophages were extracted from murine aorta and separately reanalyzed with dimensional reduction (UMAP). Right, expression of Pf4 transcript projected on the vascular tissue resident macrophage subsets UMAP plot. C Jak2 V617F WT/Flex mice were backcrossed with Pf4 Cre ± mice to generate control Pf4 Cre- Jak2 WT and Pf4 Cre + Jak2 V617F (Called Jak2 V617F Pf4) mice. D Red blood cell, white blood cell and platelet count of 7-week-old Jak2 WT and Jak2 V617F Pf4 mice ( N = 5/group). E , F representative photomicrographs and quantitative analysis of the mean aortic diameter in control 7-week-old Jak2 WT ( N = 7) and Jak2 V617F Pf4 mice ( N = 8) in the thoracic (ascending and descending) and the abdominal aorta, scale bar 1 mm. G Quantification of the collagen content (Cola1 immunostaining) in the aortic wall in 7-week-old Jak2 WT and Jak2 V617F Pf4 animals ( N = 5/group), scale bar 50 µm. H Quantification of Cola1 and Cola3 mRNA expression in aorta of 7-week-old Jak2 WT ( N = 8) and Jak2 V617F Pf4 mice ( N = 9). I Quantification of Mmp2, Mmp3, Mmp9, Mmp12, Mmp13 mRNA expression in aorta of 7-week-old Jak2 WT ( N = 8) and Jak2 V617F Pf4 mice ( N = 9). J Quantification of LYVE-1 + CD68 + tissue resident macrophages in the aorta of 7-week-old mice (Immunostaining, N = 5/group), scale bar 50 µm. K Quantification of Il6, Il1β and Tnfα mRNA expression in aorta of Jak2 WT ( N = 8) and Jak2 V617F Pf4 mice ( N = 9). L Survival curve ( N > 30/group). Data are presented as mean values ± SD. [Two-tailed Mann-Whitney test, * P < 0.05, ** P < 0.01]. Difference in survival was evaluated using log-rank test. UMAP Uniform Manifold Approximation and Projection for Dimension Reduction, Pf Platelet factor, MMP matrix metalloprotease, Il interleukin, Tnf tumor necrosis factor. Source data are provided as a Source Data file. Full size image Pharmacological activation of vascular tissue-resident macrophage activity induces dissecting aortic aneurysm in C57BL/6 mice Finally, we aimed to test a pharmacological approach in immunocompetent animals to activate in vivo vascular resident macrophages. Using an integrated dataset combining several independent single-cell studies of healthy [19] , [23] (Supplementary Fig. 12A ) and diseased mouse aortas (Supplementary Fig. 12B ), we found that the erythropoietin receptor (EpoR) was highly expressed in aortic resident macrophages. Flow cytometry analysis in different compartments confirmed that vascular resident macrophages highly and selectively expressed EPOR (Supplementary Fig. 12C ), but circulating monocytes did not. Based on these observations, we hypothesized that EPO supplementation might activate vascular tissue-resident macrophages. Eight-week-old C57BL/6 mice were treated intraperitoneally with EPO or PBS, and histological analysis of the aorta were performed after 4 weeks of treatment and survival was recorded during 7 weeks of supplementation (Supplementary Fig. 12D ). EPO treatment induced palmar erythema and polycythemia, but did not impact blood leukocyte and platelet counts (Supplementary Fig. 12E, F ). EPO treatment induced a similar vascular phenotype to that seen in JAK2V617F mutant mice, with elastin degradation (Supplementary Fig. 12G ), thinning of adventitial collagen layer (Supplementary Fig. 12H, I ), local increase in proliferating resident macrophages (Supplementary Fig. 12J, K ) and enhanced vascular pro-inflammatory responses (Supplementary Fig. 12L, M ). EPO treatment promoted aortic dilation after 4 weeks and 7 weeks (Supplementary Fig. 12N, O ), as well as aortic aneurysm (0 vs 58 %, P < 0.05) and lethal rupture (0 vs 42%, P < 0.05) (Supplementary Fig. 12P ). Pharmacological depletion of vascular tissue-resident macrophage or JAK/STAT pathway blockade attenuates aortic disease severity in JAK2V617F mutant mice Taken together, our findings provided strong evidence that JAK2V617F gain-of-function mutation in vascular tissue-resident macrophages promoted dissecting aortic aneurysm. We sought to further evaluate the effect of ablating aortic resident macrophages in the vascular wall on disease severity using Ki20227, an inhibitor of macrophage colony stimulating factor 1 (CSF1) receptor tyrosine kinase. In agreement with a previous report by Lim et al. [28] , we confirmed that Ki20227 treatment (Fig. 6A ) markedly depleted aortic macrophages (Fig. 6B, C ), but did not affect red blood cells, white blood cells and platelets in blood (Fig. 6D ). To assess the role of aortic resident macrophage depletion on aortic disease development, Ki20227 treatment was orally administered in Jak2 WT and Jak2 V617F Myel mice alternatively (Fig. 6E ) to limit long term hematopoietic toxicity (Supplementary Fig. 13A–C ). Ki20227 treatment remarkably abolished lethal aorta rupture in Jak2 V617F Myel mice (Fig. 6F ). Histological analysis performed at 15 weeks in surviving Ki20227-treated Jak2 WT and Jak2 V617F Myel mice showed that depletion of vascular tissue-resident macrophages (Fig. 6G ) abolished the pro-inflammatory signature in the mutant aorta (Fig. 6H ) and alleviated both JAKV617F -mediated aortic remodeling (Supplementary Fig. 13D ) and dilation (Fig. 6I ). Fig. 6: Pharmacological blockade of vascular tissue resident macrophage cells attenuates JAK2V617F -mediated dissecting aortopathy. A Experimental protocol of Ki20227 treatment in C57BL/6 male mice. B Immunostaining of CD68 + LYVE-1+ macrophages (Yellow) in the aorta of Ki20227- or PBS-treated mice ( N = 5/group), scale bar 50 μm. C Representative dot plot of CD45 + CD11b + Ly6G-Ly6C-CD64 + F4/80+ macrophage count in the aorta of Ki20227- or PBS-treated C57BL/6 mice. D Red blood cell, white blood cell and platelet count of Ki20227- or PBS-treated C57BL/6 mice. E experimental protocol of PBS or Ki20227 treatment in Jak2 WT and Jak2 V617F Myel mice. Jak2 WT (blue, N = 8) and Jak2 V617F Myel (Green, N = 8) mice received Ki20227 and a third group of Jak2 V617F Myel (Red, N = 12) only received control diet without pharmacological drug. F survival curve of treated mice. G Immunostaining of CD68 + LYVE-1+ macrophages (Yellow) in the aorta of surviving Ki20227-treated Jak2 WT (blue) and Jak2 V617F Myel (green) mice ( N = 8/group), scale bar 50 μm. H Quantification of Il6, Tnfα, Il1β and Ccl2 mRNA expression by RT-qPCR in the aorta of surviving Ki20227-treated Jak2 WT (blue) (N = 8 ) and Jak2 V617F Myel (green) ( N = 7) mice. I Quantitative analysis of the mean aortic diameter of surviving Ki20227-treated Jak2 WT (blue) and Jak2 V617F Myel (green) mice ( N = 8/group) in the thoracic ascending (Asc. ), thoracic descending (Desc.) and the abdominal (Abd.) aorta. J Experimental protocol describing ruxolitinib (60 mg/kg, daily during 5 weeks) or PBS treatment in Jak2 V617F HC-EC mice. K quantification of Il6, Tnfα, Il1β and Ccl2 mRNA expression by RT-qPCR in the aorta of Jak2 V617F HC-EC mice treated with PBS (Red) ( N = 10) or Ruxolitinib (Green) ( N = 8). L Quantitative analysis of the mean aortic diameter of PBS (Red, N = 7) or ruxolitinib (Green, N = 8) -treated Jak2 V617F HC-EC mice using ultrasonography in the thoracic ascending (Asc. ), thoracic descending (Desc.) and the abdominal (Abd.) aorta. M experimental protocol describing Ruxolitinib (60 mg/kg, daily during 10 weeks) or PBS treatment in Jak2 V617F Myel mice. N survival curve of treated mice ( N = 11 PBS and N = 7 Ruxolitinib). Data are presented as mean values ± SD. [Two-tailed Mann-Whitney test or Kruskal-Wallis H , I , * P < 0.05, ** P < 0.01, *** P < 0.001]. Difference in survival was evaluated using log-rank test. HC-EC, hematopoietic cells-endothelial cells; Il , interleukin; Tnf , tumor necrosis factor. Source data are provided as a Source Data file. Full size image Finally, we tested a pharmacological approach with ruxolitinib, a JAK2 inhibitor, currently used to treat JAK2V617F + patients with MPN. Jak2 V617F HC-EC and Myel mice were treated with PBS or ruxolitinib (oral gavage) daily during 5 and 10 weeks, respectively (Fig. 6 J, M). Ruxolitinib attenuated the pro-inflammatory signature of aortic wall cells with decreased mRNA expression of Il1β, Il6, Tnfα and Ccl2 in the aorta of ruxolitinib-treated Jak2 V617F HC-EC mice, compared to PBS-treated Jak2 V617F HC-EC mice (Fig. 6K ). Ruxolitinib significantly limited thoracic aorta dilation (Fig. 6L ) and decreased lethal aortic aneurysm rupture (Fig. 6N ). Here, we identified the JAK2V617F gain-of-function mutation as an independent risk factor for abnormal dilation of the ascending and descending thoracic aorta. We showed that JAK2V617F in mice drives vascular tissue-resident macrophages toward a pro-inflammatory phenotype, responsible for aortic dilation and spontaneous dissecting aortic aneurysm. Until now, little was known about the impact of JAK2V617F mutation on aortic aneurysm disease. Findings from a recently published study in angiotensin II-infused chimeric hypercholesterolemic Apoe −/ − mice, which took place while we conducted our study, agree with ours regarding the association between the JAK2V617F mutation and aortic aneurysm [29] . Yet, their experimental model was not clinically relevant and did not recapitulate the human disease. Moreover, this study did not provide any mechanistic insights into how JAK2V617F mutation can promote aortopathy and, in particular, made no mention of the central role of resident macrophages in JAK2V617F -induced severe aortopathy. In our study, using several complementary approaches, we showed that mice expressing human JAK2V617F gain-of-function mutation developed spontaneously aortic dilation at early stages and dissecting aortic aneurysm later on, in the absence of any challenge, and we identified the critical impact of JAK2V617F mutation on functions of vascular resident macrophages. Histological analysis showed increased macrophage content in the aorta of young mutant mice. Early macrophage infiltration in the aortic wall is a hallmark of aortic wall development both in mice and in humans [30] , [31] . Macrophages largely participate in aortic wall degradation and remodeling through the production of chemokines, cytokines and proteases. In animal models using angiotensin II to promote aneurysm, macrophages detected in the aneurysmal aorta were shown to mostly derive from circulating monocytes [4] , [32] , whereas in Jak2 V617F mutant mice, aortic macrophages unlikely derived from blood monocytes at early stages. At 7 weeks of age, Jak2 V617F mutant mice developed aortic dilation with no sign of infiltrating neutrophils or monocytes in the vascular wall, but with high numbers of proliferating macrophages expressing LYVE-1, a vascular tissue-resident marker. Global and single cell transcriptomic analysis confirmed that aortic macrophages in Jak2 V617F mutant mice exhibited a tissue-resident signature. Vascular tissue-resident Lyve-1 + macrophages have been shown to display protective functions against deleterious aorta remodeling in immunocompetent C57BL/6 mice [28] . In our study, we found that tissue-resident Res-MGL1 hi macrophages, abundant in Jak2 V617F Myel aortas, expressed high levels of chemokine transcripts such as Ccl2, Cxcl1, Cxcl2, Cxcl10 , as well as high levels of Nlrp3 transcripts, suggesting that JAK2V617F mutation induced a shift in macrophage profile toward a pathogenic pro-inflammatory phenotype. Increased Il1b, Il6 and Tnfα mRNA expression, as well as increased MMP activity in the aorta of 8-week-old Jak2 V617F mutant mice, likely resulted from higher content of activated macrophages in the aorta. At more advanced stages, in Jak2 V617F mutant mice with large aortic aneurysm, another dominant subset of macrophages expressing Ccr2, but not Lyve1, has been identified in the aortic wall. These Ccr2 + Lyve-1 - macrophages most likely derived from recruited blood monocytes in response to local production of chemokines, mainly Ccl2. Ccr2 is highly expressed on classical circulating monocytes and regulate their trafficking. Previous works have reported that in response to Angiotensin II infusion Ccr2 -deficient mice are characterized by decreased infiltrating monocytes in the aortic wall, decreased local inflammation and finally less severe aortic disease [33] , [34] . The JAK2V617F mutation has been shown to occur in the majority of patients with polycythemia vera [35] . The mutation also induces a polycythemia in different mouse models, due to either the proliferation and survival of erythroid progenitors carrying the mutation or local erythropoiesis in the bone marrow resulting from the release of growth factors by mutant myeloid progenitors [36] . Indirect stimulation of erythropoiesis most likely accounted for polycythemia in Jak2 V617F Myel mice since the Jak2 mutation was not detected in erythroid progenitors. Polycythemia by itself might promote arterial dilation and decrease blood pressure through the activation of the endothelial NO synthase [37] . However, we can rule out the possibility that the Jak2-associated polycythemia was responsible for aortic dilation in mutant mice since aortopathy was observed in Jak2 V617F Pf4 mice before polycythemia developed. In addition, disease severity was not affected by pharmacological correction of polyglobulia. We also found that high doses of EPO induced dissecting aortic aneurysm in immunocompetent C57BL/6 mice, supporting the critical role of the JAK2 pathway in aortic disease, but we did not specifically investigated which cell type was activated in response to EPO supplementation. Our results are in line with a recent study showing that EPO repetitive injection promoted aortic aneurysm in Apoe −/ − mice [38] . The authors found higher pro-inflammatory signature in the aorta of EPO-treated mice and suggested that endothelial cell activation might be involved in EPO-induced abdominal aortic aneurysm. However, in our study performed in normocholesterolemic mice, JAK2V617F gain-of-function mutation in vascular cells, and specifically in endothelial cells, did not promote aortic disease. The relevance of our results in experimental murine models to the human situation are supported by the present finding of aortic dilation in patients with JAK2V617F mutation. In addition, several case reports also described arterial aneurysms in patients with JAK2 + myeloproliferative neoplasm [39] , [40] . More recently, in a genome-wide association study (GWAS) using the UK Biobank, an intronic variant located within the gene encoding JAK2 tyrosine kinase has been linked to aortic aneurysm [41] . Conversely to what we observed in Jak2 V617F mutant mice, dissecting aortic aneurysm is not common in JAK2V617F + patients. This discrepancy could be explained by the fact that JAK2V617F mutation in human is a somatic mutation occurring at late stages in adult whereas it is a germline mutation in mice who developed severe hematological disease at early stages of life. In addition, this discrepancy between human and mice data might be accounted for by the vascular protection by specific drugs, such as ruxolitinib, that are currently used to treat JAK2V617F + myeloproliferative diseases. Interestingly, in our study, we showed that ruxolitinib attenuated pro-inflammatory signature in the aortic wall and protected against deleterious aortic remodeling and lethal rupture. The protection induced by Ki20227 treatment supports the role of resident vascular macrophages in the pathophysiology of JAK2V617F-mediated aortopathy. However, Ki20227 could have off-target effects, such as angiogenesis inhibition [42] . However, in our mutant models, we did not find any evidence that JAK2V617F mutation impaired angiogenesis in the aortic wall. Human samples analysis We screened in a cohort of JAK2V617F + patients treated in Saint-Antoine Hospital (Assistance Publique-Hôpitaux de Paris), those who had a thoraco-abdominal CT-scan during the last 5 years. Controls were gender- and age-matched patients hospitalized in non-hematology department (Saint-Antoine Hospital) and who had a thoraco-abdominal CT-scan during the same period. Cardiovascular risk factors were recorded and used for multivariate adjustment. Aorta measurements were performed by two radiologists worked on the original axial data sets and used electronic calipers to measure the largest diameter of aorta at three points: (1) the mid ascending aorta at the level of the right pulmonary artery, (2) the mid descending aorta at the level of the aortic valve and (3) the maximal infrarenal aortic diameter. In order to evaluate the effect of the JAK2V617F mutation on the aorta diameter, we perfomed both univariate and multivariate logistic regression. Classical risk factors of aortic aneurysm such as age, arterial hypertension, diabetes, smoking status and gender was included in the multivariate logistic regression. The aorta was considered as dilated if diameter was higher than the average of the whole included patients. Written informed consent was not required, in compliance with French law on retrospective studies of anonymized data (loi Jardé, MR004). All local medico-administrative data bases are declared to the general register of data processing of the Assistance publique-Hopitaux de Paris (Bureau de la protection des données, France no. 20220106150715). Murine models Experiments were conducted according to the guidelines formulated by the European Community for experimental animal use (L358-86/609EEC) and approved by the Ethical Committee of INSERM CEEA34 (MESR26963) and the French Ministry of Agriculture (agreement A75-15-32). Mouse breeding occurred in our animal facility in accordance with local recommendations. Animals were provided with food and water ad libitum. All the animals were maintained under identical standard conditions (housing, regular care and normal chow). Mice were maintained in isolated ventilated cages under specific pathogenfree conditions. Before euthanasia by cervical dislocation, animals were anesthetized with isoflurane (3% in oxygen). Control mice were matched with littermates of the appropriate, age, sex, and genetic background to account for any variation in data. All mice were on a C57BL/6 background. Jak2 V617F HC-EC mice were obtained by crossing VE-cadherin-Cre [15] (Jackson Laboratory) transgenic mice with Jak2V617F Flex/WT mice [43] . Jak2 V617F HC-EC mice have been generated by PE Rautou’s group [16] . Jak2 V617F EC mice were obtained by crossing VE-Cadherin-cre-ERT2 transgenic mice (Provided by R.H. Adams, Max Planck Institute for Molecular Biomedicine, Münster, Germany) [44] with Jak2V617F Flex/WT mice. Jak2 V617F Myel mice were obtained by crossing LysM-Cre transgenic mice (Jackson Laboratory) with Jak2V617F Flex/WT mice. Jak2 V617F Pf4 mice were obtained by crossing Pf4 -Cre transgenic mice [45] , [46] with Jak2V617F Flex/WT. In all experiments, male and female mice were used. For induction of Cre recombinase expression in Jak2V617F Flex/WT; VE-Cadherin-creERT2 mice, mice were injected intraperitoneally with tamoxifen (Sigma, T5648), 1 mg/mouse/day for 5 consecutive days over 2 consecutive weeks (10 mg in total per mouse) between the age of 5 to 7 weeks. The Flex (Flip-Excision) strategy allows expression of a mutated gene in adulthood, in a temporal and tissue-specific manner [47] . Bone marrow transplantation Six to 8-week-old C57BL/6 J and Jak2 V617F HC-EC mice were subjected to medullar aplasia following sublethal total body irradiation (9.5 grays). At day 1, irradiated mice were repopulated intravenously with bone marrow cells (10 millions) isolated from femurs and tibias of age matched Jak2 V617F HC-EC and C57BL/6 J CD45.1 or CD45.2 control mice. Mice were followed-up during 1–3 months with repetitive blood cells analysis and aortic diameter measurements by echography. Blood cell count analysis Blood was collected through the mandibular vein in a tube pre-coated with EDTA after transient anesthesia (Isoflurane). Blood counts analyses were performed using a Hemavet 950FS analyser (Drew scientific). Fluorescence molecular tomography (FMT) imaging Twenty-four hours before sacrifice, Jak2 V617F HC-EC and Jak2 V617F Myel animals were anesthetized with isoflurane and received 150 μL intravenously of a fluorescent imaging probe MMPsense 680 (NEV 10126, PerkinElmer). The probe is optically silent in its unactivated state and becomes highly fluorescent following activation by MMPs including MMP-2, −3, −9, and −13. Images were acquired using a fluorescence molecular imaging system (FMT 2500TM, VisEnMedical). In vivo treatment Erythropoietin (Eprex, Janssen) (EPO) was administered for 5 and 7 consecutive weeks by intraperitoneal injection to 8-week-old C57BL/6 males (5000 UI/kg, 3 times per week). EPO was prepared in PBS. Control mice received the same volume of vehicle (PBS). Ruxolitinib (Jakavi, Novartis) was administered for 5 consecutive weeks (30 mg/kg, 2 times per day) by oral gavage to Jak2 V617F HC-EC . Ruxolitinib was prepared from 10 mg commercial tablets in PEG300/5% dextrose mixed at a 1:3 ratio. Control mice were administered the same volume of vehicle (PEG300/5% dextrose). Five-week-old C57BL/6 mice received daily oral administration of Ki20227 [9] by food for 2 weeks. 5-week-old Jak2 V617F Myel mice were alternatively fed with Ki20227 and chow diet for 10 weeks. Phenylhydrazine (PHZ) was administered every 3 days by intra peritoneal injection to 6-week-old Jak2 V617F HC-EC mice (25 mg/kg body weight). PHZ was prepared in PBS and control mice received the same volume of vehicle. Histological analysis The aorta was flushed with cold PBS through the left ventricle and removed from the root to the iliac bifurcation. Abdominal aorta was used for histologic studies. The suprarenal region of the abdominal aorta, subjected to aneurysmal development, was harvested and embedded in both cryostat and paraffin and 7-μm thick sections were used for histology and immunohistochemistry analysis. Sections were stained with Orcein (MMFrance) for detection of elastin layers. The mean number of elastin layers was quantified by a researcher blinded to the experimental protocol (4 measurements/section, 8 sections/mouse). Sections were stained for macrophages using a rat anti– mouse CD68 primary antibody (MCA1957, clone FA-11, Bio Rad) revealed with an anti–rat Cy5 secondary antibody (712-175-153, Jackson ImmunoResearch). The percentage of cellular area positive for CD68 staining (macrophages) was quantified using Histolab software (Microvision) and the CD68 + area/total aortic wall area (media + adventitia) ratio was calculated. For resident macrophages, sections were also stained with a rabbit anti-mouse LYVE-1 (ab33682, polyclonal, Abcam) revealed with an anti–rabbit Cy3 secondary antibody (711-165-152, Jackson ImmunoResearch). Total macrophages (CD68 + ) and resident macrophages (CD68 + LYVE-1 + ) were manually counted (8 sections per mouse for each experiment). Proliferative macrophages were stained with a rabbit anti-mouse Ki67 (RM-9106-S, clone SP6, Epredia) after fixation and permeabilization (Triton 0.01%) and revealed with an anti–rabbit Cy3 secondary antibody (711-165-152, Jackson ImmunoResearch). Total macrophages (CD68 + ) and proliferative macrophages (CD68 + Ki67 + ) were manually counted. The media was stained with a rabbit anti-mouse Alpha Smooth muscle actin (ab5694, polyclonal, abcam) after fixation and permeabilization (Triton 0.01%) and revealed with an anti–rabbit Cy3 secondary antibody (711-165-152, Jackson ImmunoResearch). The quantification was obtained by calculating the aSMA positive area and the total media area using Histolab software (Microvision) and the aSMA+ area/total media ratio was calculated. The adventital collagen was stained with a rabbit anti-mouse Collagen Type I (234167, polyclonal, Merck Millipore) revealed with an anti–rabbit Cy5 secondary antibody (711-175-152, Jackson ImmunoResearch). Total advential collagen positive area was calculated using ImageJ (NIH) software. In each experiment, 8 sections per mouse were quantified. Histology quantifications were done by a researcher blinded to the experimental protocol. Epifluorescence analysis, brightfield and polarized light imaging were done using Leica DM6000B microscope. Flow cytometry FACS analysis was performed on total aortas. The day of sacrifice, animals were perfused with cold PBS and whole aortas were rapidly cleaned and harvested under a dissection microscope. Aortas were minced and incubated 30 min at 37 °C in an enzymatic digestion cocktail (Collagenase I (450 U/ml, Sigma Aldrich), Collagenase XI (125 U/ml, Sigma Aldrich), Hyaluronidase (60 U/ml, Sigma Aldrich), DNAse (60 U/ml, Sigma Aldrich) and Elastase (0.372 U/ml, Sigma Aldrich). Then a mechanic digestion was performed to pass the cells through a 100 µm filter before the staining. Leukocyte suspension was obtained from aorta and extracellular antigens were stained with fluorescent labeled anti-mouse antibodies for 30 min at 4 °C. Flow cytometric acquisitions were done on a BD LSRFortessa (BD Biosciences) and data were analyzed using FlowJo Software (TreeStar, Inc.). Forward scatter (FSC) and side scatter (SSC) were used to gate live cells, red blood cells, debris, cell aggregates and doublets being excluded. Lymphocytes T were identified as CD45 + /CD11b-/CD3 + ; Lymphocytes B as CD45 + /CD11b-/B220 + ; Neutrophils as CD45 + /CD11b + /Ly6G + ; Monocytes as CD45 + /CD11b + /Ly6G-/Ly6C + ; Macrophages as CD45 + /CD11b + /Ly6G-/F4/80 high /CD64 high ; Resident macrophages as CD45 + /CD11b + /Ly6G-/F4/80 high /CD64 high /Lyve-1 + ; Dendritic cells were CD45 + /CD11c high /CMHII high . The following primary conjugated antibodies were used for staining in the aorta: anti-CD45 (Alexa Fluor 700, clone 30-F11, BD Biosciences), anti-CD11b (BV605, clone M1/70, BD Biosciences), anti-Ly6C (APC-Cy7, clone AL-21, BD Biosciences), anti-Ly6G (BUV395, clone 1A8, BD Biosciences), anti-CD64 (BV421, clone X54-5/7.1 Biolegend), anti-F4/80 (PE, clone CI:A3-1, Abcam), anti-CD11c (PerCP-Cy5.5, clone HL3, BD Biosciences), anti-MHC-II (BV510, clone M5/114.115.2, BD Biosciences), anti-CD3 (PE-Cy7, clone 145-2C11, BD Biosciences), anti-CD45R (B220) (BUV496, clone RA3-6B2, BD Biosciences), anti-LYVE1 (clone ALY7, Life Technologies), anti-EPO-R (PE, polyclonal, Clinisciences), anti-CD45.1 (BV605, clone A20, Biolegend), anti-CD45.2 (BV510, clone 104, Biolegend). The following primary conjugated antibodies were used for the staining in the peritoneal macrophages and in the bone marrow: anti-CD45 (Alexa Fluor 700, clone 30-F11, BD Biosciences), anti-CD11b (BV605, clone M1/70, BD Biosciences), anti-Ly6C (APC-Cy7, clone AL-21, BD Biosciences), anti-Ly6G (BUV395, clone 1A8, BD Biosciences), anti-CD64 (BV421, clone X54-5/7.1 Biolegend), anti-F4/80 (FITC, clone BM8-1, Tonbo), anti-LYVE-1 (clone ALY7, Life Technologies), anti-EPO-R (PE, polyclonal, Clinisciences). Determination of JAK2V617F allele burden on bone marrow hematopoietic cells Femur and tibia from control Jak2 WT and Jak2 V617F HC-EC mice were crushed and filtered in PBS + EDTA 2 mM+FBS 2%. Mature erythroid cells were then lysed in an ammonium buffer. For progenitor cells analysis, an enrichment in CD117 + (Kit + ) cells was performed by magnetic cell sorting using anti-CD117 microbeads according to manufacturer’s instruction (Miltenyi Biotec). Cells were then labeled 30 min at 4 °C with the following antibodies: for progenitors cells: Biotin-Lin (mix of anti-CD4, CD5, CD8a, Mac-1, B220, Ter119, Gr-1 antibodies, all from BD Bioscience); Kit APC (Biolegend # 105812); Sca 1 BV421 (Biolegend #108128); CD41 APC-Cy7 (Biolegend #133928); CD34 FITC (Biolegend #553733); CD16/32 BV510 (Biolegend #101333) for precursors and mature cells: CD41 APC-Cy7 (Biolegend #133928); Ter119 PE-Cy7 (Biolegend #116222); Gr1 FITC (Biolegend #108406); CD3 PE (Biolegend #100206); CD19 PB (Biolegend #115523). After washing, Steptavidine PerCP-Cy5.5 was added during 15 minutes at 4 °C and cells were then sorted on a FACS Aria LSR (Becton Dickcinson). The following populations were isolated: LSK (Lin- Kit+ Sca + ); Megakaryocytes-Erythroid Progenitors (MEP) (Lin- Kit+ Sca- CD CD34-CD16/32-41-); Granulocyte-Monocyte Progenitors (GMP): Lin- Kit+ Sca- CD41- CD34 + CD16/32 + ; Megakaryocytic progenitors (MkP, Lin- Kit+ Sca- CD41 + ); T Lymphocytes (CD3 + ); B Lymphocytes (CD19 + ); Granulocytic precursors (CD19-CD3-Gr1 + ); Erythroid precursors (CD19-CD3-Ter119 + ). Cells were frozen at −80 °C and DNA extracted using Nucleospin Tissue extraction kit (Macherey Nagel). The JAK2V617F allele burden was determined using a droplet digital PCR technic (Biorad QX200 system). The following primer and probes were used: mJAK2-FwdCGAAGCAGCAAGCATGATGAG mJAK2-RevGAGAGTAAGTAAAGCCAcCTGCT mJAK2-Probe WTHEX-ATTATGGTGTCTGTGTCTGTGGAG-BHQ Fwd mJAK2 ddPCRAAGCCCAGGTGATGGATGAGG Rev mJAK2 ddPCRGTTACACGAGTCACCCATAATC Probe mJAK2V617F ddPCRFAM-TACGAAGTTATTGGATTTCCTGCG-BHQ The amplification program was as follows: 95 °C during 10′, before 40 cycles at 94 °C during 30′ and 57 °C during 1′, and a final step at 98 °C during 10′. Results were analyzed with Quantasoft software and expressed as the proportion of mutated allele among the number of copies of total JAK2 detected. Bulk RNA sequencing & analysis After RNA extraction, RNA concentrations were obtained using nanodrop or a fluorometric Qubit RNA assay (Life Technologies, Grand Island, New York, USA). The quality of the RNA (RNA integrity number) was determined on the Agilent 2100 Bioanalyzer (Agilent Technologies, Palo Alto, CA, USA) as per the manufacturer’s instructions. To construct the libraries, 100 ng of high quality total RNA sample (RIN > 8) was processed using NEBNext Ultra II RNA Library Prep Ki (New England BioLabs) according to manufacturer instructions. Briefly, after purification of poly-A containing mRNA molecules, mRNA molecules are fragmented and reverse- transcribed using random primers. Replacement of dTTP by dUTP during the second strand synthesis will permit to achieve the strand specificity. Addition of a single A base to the cDNA is followed by ligation of Illumina adapters. Libraries were quantified by qPCR using the KAPA Library Quantification Kit for Illumina Libraries (KapaBiosystems, Wilmington, MA) and library profiles were assessed using the DNA High Sensitivity LabChip kit on an Agilent Bioanalyzer. Libraries were sequenced on an Illumina Nextseq 500 instrument using 75 base-lengths read V2 chemistry in a paired-end mode. After sequencing, a primary analysis based on AOZAN software (ENS, Paris) was applied to demultiplex and control the quality of the raw data (based of FastQC modules/version 0.11.5). Obtained fastq files were then aligned using STAR algorithm (version 2.5.2b) and quality control of the alignment realized with Picard tools (version 2.8.1). Reads were then counted using Featurecount (version Rsubread 1.24.1) and the statistical analyses on the read counts were performed with the DESeq2 package version 1.14.1 to determine the proportion of differentially expressed genes between two conditions. Raw fastq files were mapped to mouse genome GRCm38 release 96 with STAR 2.7.1a (Spliced Transcripts Alignment To a ref. 48 . Normalization and differential expression analysis was performed with DESeq2 1.32.0 package ( https://doi.org/10.1186/s13059-014-0550-8 ). Adjusted p -values were calculated using Benjamini and Hochberg’s approach, and genes with adjusted p -value <0.05 were considered as differentially expressed and selected for functional enrichment using clusterProfiler package v4.0.5 ( https://doi.org/10.1093/bioinformatics/btq064 ). CITE-seq Jak2 WT ( n = 5) and Jak2 V617F Myel ( n = 5) mice under isoflurane anesthesia received 2 µg of anti-CD45.2-APC (clone 104, BioLegend) i.v. 5 min before sacrifice to label circulating immune cells [19] and were killed by cervical dislocation. Upon collection of the aorta using a stereomicroscope, aneurysm development was macroscopically detected in 2 Jak2 V617F Myel mice. Aortas were collected and enzymatically digested in RPMI medium containing 450 U/ml collagenase I (Sigma-Aldrich C0130), 125 U/ml collagenase XI (Sigma-Aldrich C7657), 60 U/ml Hyaluronidase (Sigma-Aldrich H3506) and 60U/ml DNAse1 (Roche #11284932001) for 45 min at 37 °C with agitation, washed in PBS + 1% FCS and passed through a 70 µm cell strainer. After washing in PBS + 1%FCS, aortic cells were resuspended in erythrocyte lysis buffer (ACK buffer) for 5 min and washed again with PBS + 1% FCS. Cells were plated in round bottom 96 well plates, and incubated for 10 min on ice with anti-CD16/32 (BioLegend, Clone 93, 10 µg/ml in PBS + 1% FCS) to block unspecific binding of antibodies to Fc receptors. Cells were subsequently labeled in a final volume of 60 µl for 25 minutes at 4 °C with a mix containing CITE-seq [20] antibodies (TotalSeq-A, BioLegend, see table below), 1:1000 Fixable Viability Dye e780 (ThermoFisher Scientific 65-0865-14), 2 µg/ml anti-CD45.2 BV421 ( Jak2 WT samples) or 2 µg/ml anti-CD45.2 Alexa488 ( Jak2 V617F samples). Each unique sample was labeled with a specific Hashtag antibody for cell hashing [49] (Hashtag 1 to 5: Jak2 WT aortas, Hashtag 7 and 9: Jak2 V617F Myel with aneurysm; Hashtag 6, 8, and 10: Jak2 V617F Myel without aneurysm; final concentration 1:100, BioLegend TotalSeq-A). TotalSeq-A antibody against: BioLegend Cat# Dilution Ly6G 127655 500 CD11b 101265 500 CD62L 104451 500 IA_IE 107653 500 CD54 (ICAM1) 116127 500 Ly6C 128047 800 CD115 135533 500 CXCR4 146520 500 Msr1 154703 500 CD64 139325 500 FCeRIa 134333 500 CCR3 144523 500 CD49d 103623 500 CD80 104745 500 CD117 105843 500 Sca1 108147 500 CD11c 117355 500 TIM4 130011 500 CX3CR1 149041 500 XCR1 148227 500 F4/80 123153 500 CD86 105047 500 CD135 135316 500 CD103 121437 500 CD169 142425 500 CD8a 100773 500 SiglecH 129615 500 CD19 115559 500 CD3 100251 500 CD63 143915 500 CD9 124819 500 CD163 155303 500 NK1.1 108755 500 CD127 135045 500 CD68 137031 500 Sirpa 144033 500 ITGB7 321227 500 CD4 100569 500 CD26 137811 500 MGL2 146817 500 TCRgd 118137 500 CCR2 150625 500 CD44 103045 500 CD21/35 123427 500 CD43 143211 500 Armenian Hamster IgG Isotype Ctrl 400973 500 Rat IgG1, κ Isotype Ctrl 400459 500 Rat IgG2a, κ Isotype Ctrl 400571 500 Rat IgG2b, κ Isotype Ctrl 400673 500 CD47 127535 500 SiglecF 155513 500 CD137 106111 500 CD36 102621 500 CCR5 107019 500 CD278 117409 500 PIR-A_B 144105 500 CD5 100637 500 CD304 145215 500 CD40 124633 500 CD14 123333 500 CD95 152614 500 CD300c_d 148005 500 IL1RL1 145317 500 TCRbeta 109247 500 Mac2 125421 500 CD137L 107109 500 CD178 106613 500 CD55 131809 500 CD226 128823 500 TIGIT 142115 500 CD39 143813 500 JAML 128507 500 CXCR5 145535 500 MGL1 145611 500 CD24 101841 500 After labeling, cells were washed twice in PBS + 1% FCS and pooled. Viable leukocytes were sorted with exclusion of contaminating circulating leukocytes (CD45.2-APC + ) using a BD FACS Aria III with a 100 µm nozzle. 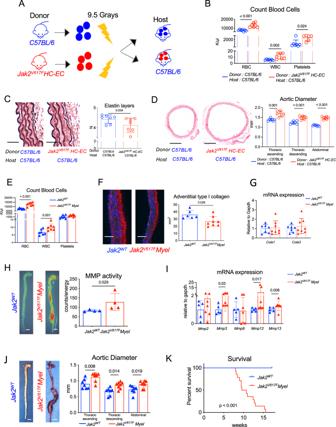Fig. 2: JAK2V167F mutation in hematopoietic cells promoted dissecting aortopathy. AExperimental protocol of WT orJak2V617FHC-ECbone marrow cell transplantation in lethally irradiatedC57BL/6mice (7/Group).BRed blood cell, white blood cell and platelet count of 20-week-old chimeric mice (N= 7/group).CQuantification of the number of elastin layers in the aortic wall by Orcein staining at sacrifice (N= 7/group), scale bar 50 μm.DRepresentative photomicrographs and quantitative analysis of the mean aortic diameter in WT orJak2V617FHC-ECchimeric mice (N= 7/group) in the thoracic (ascending and descending) and the abdominal aorta, scale bar 0.5 mm.ERed blood cell, white blood cell and platelet count of 7-week-oldJak2WTand Jak2V617FMyelmice (N= 7/group).FQuantification of the collagen content (Cola1 immunostaining) in the aortic wall in 7-week-oldJak2WT(N= 6) andJak2V617FMyelanimals (N= 8), scale bar 50 μm.GQuantification ofCola1andCola3mRNA expression in aorta of 7-week-oldJak2WT(N= 7) andJak2V617FMyelmice (N= 8).HFluorescent Molecular Tomography quantification of matrix metalloproteinase (MMP-2, −3, −9, and −13) activity in aorta of 9-week oldJak2WTandJak2V617FMyelmice (N= 4/group), scale bar 1 mm. I, quantification ofMmp2, Mmp3, Mmp9, Mmp12, Mmp13mRNA expression in aorta of 7-week-oldJak2WT(N= 5) andJak2V617FMyelmice (N= 7).JRepresentative photomicrographs and quantitative analysis of the mean aortic diameter in 7-week-oldJak2WT(N= 7) andJak2V617FMyel(N= 8)mice in the thoracic (ascending and descending) and the abdominal aorta, scale bar 1 mm.KSurvival curve ofJak2WT(N= 11) andJak2V617FMyelmice (N= 14). Data are presented as mean values ± SD. [Two-tailed Mann-Whitney test, *P< 0.05, **P< 0.01, ***P< 0.001]. Difference in survival was evaluated using log-rank test. HC-EC, hematopoietic cells-endothelial cells; MMP, matrix metalloprotease. Source data are provided as a Source Data file. The amount of sorted cells was adjusted so that cells from Jak2 WT (CD45.2-BV421 + ) and from Jak2 V617F aortas (CD45.2-Alexa488 + ) each represented ~50% of the total sorted cells. Cells were sorted in PBS supplemented with 1% PBS, and washed twice post-sort in PBS + 0.04% UltraPure BSA (ThermoFisher AM2616). Cells were counted in Trypan blue to assess viability (>80%). A total of 20,000 cells were loaded at a concentration of 500 cells/µl in the 10× Genomics Chromium (Single Cell 3′ v3 reagents, 10× Genomics) and scRNA-seq, ADT and HTO libraries prepared and sequenced as described in [26] . Single-cell RNA-seq data analysis A total of 10× Genomics data, including HTO and ADT libraries, was demultiplexed using Cell Ranger software (Pipeline Version 6.0.2). Mouse mm10 reference genome was used for the alignment and counting steps. The Feature-Barcode matrix obtained from Cell Ranger was further analyzed in Seurat v3.1.1 [50] . The “HTODemux” function was used to identify sample of origin of single cells, exclude multiplets (i.e. cells positive for more than one hashtag signal) and cells with no detectable hashtag signal. Cells with more than 10% mitochondrial transcripts were excluded from further analysis. Data were normalized using the “NormalizeData” function, and 2000 variable features identified with the “FindVariableFeatures” function using the “vst” selection method. Data were scaled using the “ScaleData” function and principal component (PC) analysis performed. Clustering was performed using the “FindNeighbors” and “FindClusters” functions with 20 PCs and a resolution parameter of 0.3. Uniform Manifold Approximation and Projection (UMAP) dimensional reduction was performed using 20 PCs. Immune cell populations were identified based on CITE-seq signal for established cell surface markers (see Results). Cells corresponding to monocytes/macrophages were subset in a new Seurat object and reclustered. This refined analysis revealed clusters of monocyte/macrophages with very low RNA content that were considered as low quality/dead cells and removed from further analysis. The curated monocyte/macrophage dataset was analyzed with clustering (resolution 0.8) and dimensional reduction as described above. 2 clusters of Ccr2 + macrophages with a clearly overlapping pro-inflammatory gene expression profile were manually pooled into the “ Ccr2 + Inflammatory” macrophage cluster. Enriched transcripts and cell surface markers in monocyte/macrophage populations were determined using the “FindAllMarkers” function. Data visualizations were generated using built-in functions in Seurat (e.g. “FeaturePlot”, “DotPlot”) and dittoSeq ( https://github.com/dtm2451/dittoSeq ). Quantitative real-time polymerase chain reaction Thoracic aortas were harvested after flushing with cold PBS and were frozen at −80 °C. Total RNA was extracted from frozen mouse thoracic aorta samples with Qiagen columns (RNeasy MiniSpin Columns) using a polytron (T25 basic, IKA, Labortechnik). The phase containing RNAs was then recuperate and washed with molecular biology water. 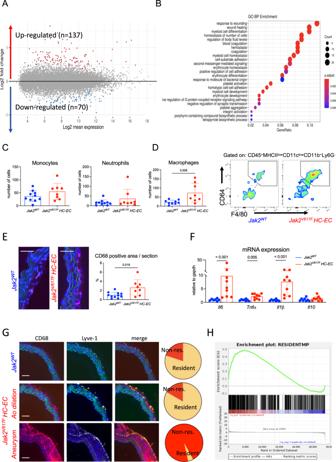Fig. 3: JAK2V167F mutation induces pro-inflammatory signature in the aortic wall. ADifference in gene expression in the aorta of 7-week-oldJak2WT(N= 4) andJak2V617FHC-ECmice (N= 3).BTop Gene Ontology terms mostly enriched among genes upregulated in the aorta ofJak2V617FHC-ECmice when compared toJak2WTmice.CFlow cytometry quantification of CD45 + CD11clowCMHIIlowCD11b + Ly6G-F4/80lowCD64lowLy6C + monocytes and CD45 + CD11clowCMHIIlowCD11b + Ly6G+ neutrophils in the aorta of 7-week-oldJak2WT(N= 10) andJak2V617FHC-ECanimals (N= 8).DFlow quantification and representative dot plot of CD45 + CD11clowCMHIIlowCD11b + Ly6G-F4/80highCD64highmacrophage count in the aorta of 7-week-oldJak2WT(N= 10) andJak2V617FHC-ECanimals (N= 8).EQuantification and representative photomicrographs of CD68 positive macrophages in the aorta of 7-week-old mice (N= 11 in control group andN= 8 inJak2V617FHC-ECgroup), scale bar 50 µm.FQuantification ofIl6, Tnfα, Il1β,andIl10mRNA expression by RT-qPCR in the aorta of 7-week-oldJak2WT(N= 8) andJak2V617FHC-ECanimals (N= 9).GImmunofluorescence staining in the aortic wall ofJak2WTandJak2V617FHC-ECmice, DAPI (Blue), CD68 (Red), LYVE-1 (Green), scale bar 50 μm. resident macrophages were defined as CD68 + LYVE-1+ cells (N= 5/group).HGSEA for genes related to a gene set signature for tissue resident macrophage19in the aorta of 7-week-oldJak2WTandJak2V617FHC-ECanimals (N= 4/group). Data are presented as mean values ± SD. [Two-tailed Mann-Whitney test, *P< 0.05, **P< 0.01, ***P< 0.001]. HC-EC, hematopoietic cells-endothelial cells;Il, interleukin;Tnf, tumor necrosis factor; GSEA, gene set enrichment analysis. Source data are provided as a Source Data file. RNA quality control and concentration were performed using Nanodrop 2000 (Thermofisher scientific). and then stored at −80 °C. Reverse transcription was done following manufacturer instruction (kit QuantiTect Reverse Transcription (Qiagen)). Real-time fluorescence monitoring was performed with the Applied Biosystems, Step One Plus Real-Time PCR System with Power SYBR Green PCR Master Mix (Eurogentec). qPCR was performed in triplicate for each sample. 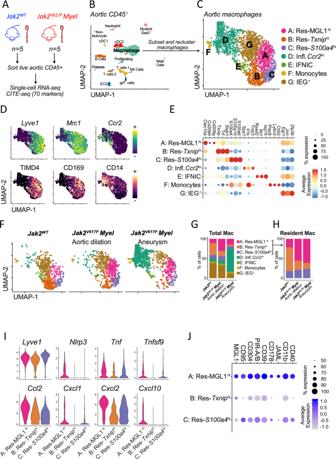Fig. 4:Jak2V617FMyelaortas harbor pro-inflammatory Lyve1 + tissue resident macrophages. AExperimental design,BUMAP visualization of scRNA-seq profiles of CD45 + cells extracted fromJak2WTandJak2V617FMyelaortas.CSingle-cells annotated as macrophages on the UMAP displayed in B were in silico extracted, reanalyzed with dimensional reduction (UMAP) and clustered identifying 7 major populations (Annotated A to G).DExpression intensity of transcripts (top) and cell surface markers (bottom) characteristic of tissue resident macrophages (Lyve1, Mrc1, TIMD4, CD169) and recruited monocytes/macrophages (Ccr2, CD14) projected on the macrophage UMAP plot.EExpression of selected marker transcripts in the 7 macrophage populations.FMacrophage UMAP plot split according to experimental condition (color code as inB).GProportions of macrophage populations among total aortic macrophages.HProportions of tissue resident macrophage subsets among total aortic tissue resident macrophages.INormalized expression of the indicated transcripts in tissue resident macrophage subpopulations.JAverage expression of the indicated cell surface markers (measured by CITE-seq) in tissue resident macrophage subpopulations. UMAP, Uniform Manifold Approximation and Projection for Dimension Reduction,scsingle cell,CITE-seqCellular Indexing of Transcriptomes and Epitopes by Sequencing. GAPDH cycle threshold was used to normalize gene expression: (F: 50 -CGTCCCGTAGACAAAATGGTGAA-30; R: 50 - GCC GTGAGTGGAGTCATACTGGAACA-30). Relative expression was calculated using the 2-delta-delta CT method followed by geometric average, as recommended. The following primer sequences were used: Il1β: Forward 5′-GAAGAGCCCATCCTCTGTGA-3′; Reverse 5′-GGGTGTGCCGTCTTTCATTA-3′; Tnfα: Forward 5′-GATGGGGGGCTTCCAGAACT-3′, Reverse: 5′-CGTGGGCTACAGGCTTGTCAC-3′, Il6: Forward 5′-TGACAACCACGGCCTTCCCTA-3′, Reverse 5′-TCAGAATTGCCATTGCACAACTCTT-3′, Il10: Forward 5′-CTCCTAGAGCTGCGGACTGCCTTCA-3′, Reverse 5′-CTGGGGCATCACTTCTACCAGGTAAAA-3′, Ccl2: forward 5′-CCCCACTCACCTGCTGCTA-3′, reverse 5′-TACGGGTCAACTTCACATTCAAA-3′ Blood pressure Non-invasive systolic and diastolic blood pressure monitoring using tail cuff was done using Visitech BP-2000. Mice were trained for blood pressure 2 days prior to taking readings. Blood pressures were measured at 7-week-old. In each animal, the system automatically performed 4 measurements first, which were not recorded, then 10 consecutive measurements that were recorded. Ultrasound study We used Vevo 2100 ultrasound imager (VisualSonics) equipped with MS550D 22–55 MHz transducer. During imaging, each mouse was anesthetized with 2% isoflurane administered through an adapted nose cone. The mouse was then placed in a supine position on a heated platform to maintain its body temperature at approximately 37 °C. The hair over the areas being imaged was removed with a depilatory cream. Degassed ultrasound gel was used as a coupling medium. The ultrasound device was placed on the thorax and then on the abdomen of the mouse. Sagittal and transversal images were acquired. 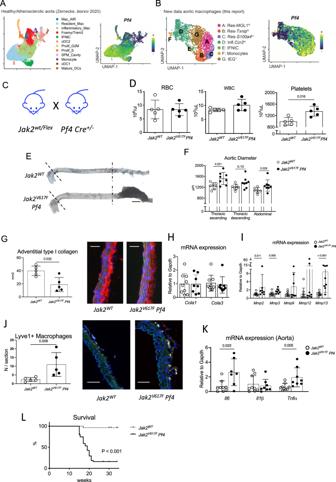Fig. 5: JAK2 mutation in vascular tissue resident macrophage cells promotes dissecting aortopathy. ALeft, cells corresponding to monocytes/macrophages/dendritic cells were extracted from murine healthy and atherosclerotic plaques and separately reanalyzed with dimensional reduction (UMAP)25. Right, expression ofPf4transcript projected on the vascular monocytes/macrophages/dendritic cells UMAP plot.BLeft, cells corresponding to macrophages were extracted from murine aorta and separately reanalyzed with dimensional reduction (UMAP). Right, expression ofPf4transcript projected on the vascular tissue resident macrophage subsets UMAP plot.CJak2V617FWT/Flexmice were backcrossed withPf4 Cre± mice to generate controlPf4Cre-Jak2WTandPf4 Cre+Jak2V617F(Called Jak2V617FPf4)mice.DRed blood cell, white blood cell and platelet count of 7-week-oldJak2WTand Jak2V617FPf4mice (N= 5/group).E,Frepresentative photomicrographs and quantitative analysis of the mean aortic diameter in control 7-week-oldJak2WT(N= 7) andJak2V617FPf4mice (N= 8) in the thoracic (ascending and descending) and the abdominal aorta, scale bar 1 mm.GQuantification of the collagen content (Cola1 immunostaining) in the aortic wall in 7-week-oldJak2WTand Jak2V617FPf4animals (N= 5/group), scale bar 50 µm.HQuantification ofCola1andCola3mRNA expression in aorta of 7-week-oldJak2WT(N= 8) andJak2V617FPf4mice (N= 9).IQuantification ofMmp2, Mmp3, Mmp9, Mmp12, Mmp13mRNA expression in aorta of 7-week-oldJak2WT(N= 8) andJak2V617FPf4mice (N= 9).JQuantification of LYVE-1 + CD68 + tissue resident macrophages in the aorta of 7-week-old mice (Immunostaining,N= 5/group), scale bar 50 µm.KQuantification ofIl6, Il1βandTnfαmRNA expression in aorta ofJak2WT(N= 8) andJak2V617FPf4mice (N= 9).LSurvival curve (N> 30/group). Data are presented as mean values ± SD. [Two-tailed Mann-Whitney test, *P< 0.05, **P< 0.01]. Difference in survival was evaluated using log-rank test.UMAPUniform Manifold Approximation and Projection for Dimension Reduction,PfPlatelet factor,MMPmatrix metalloprotease,Ilinterleukin,Tnftumor necrosis factor. Source data are provided as a Source Data file. 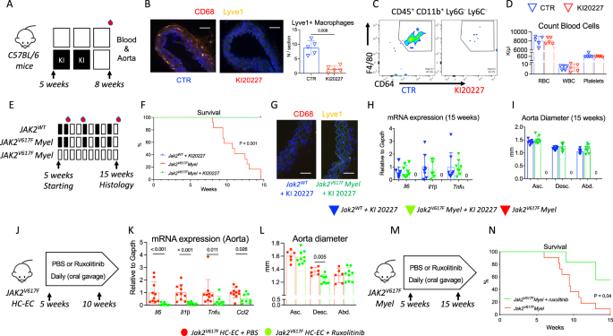Fig. 6: Pharmacological blockade of vascular tissue resident macrophage cells attenuatesJAK2V617F-mediated dissecting aortopathy. AExperimental protocol of Ki20227 treatment inC57BL/6male mice.BImmunostaining of CD68 + LYVE-1+ macrophages (Yellow) in the aorta of Ki20227- or PBS-treated mice (N= 5/group), scale bar 50 μm.CRepresentative dot plot of CD45 + CD11b + Ly6G-Ly6C-CD64 + F4/80+ macrophage count in the aorta of Ki20227- or PBS-treatedC57BL/6mice.DRed blood cell, white blood cell and platelet count of Ki20227- or PBS-treatedC57BL/6mice.Eexperimental protocol of PBS or Ki20227 treatment inJak2WTandJak2V617FMyelmice.Jak2WT(blue,N= 8) andJak2V617FMyel(Green,N= 8) mice received Ki20227 and a third group ofJak2V617FMyel(Red,N= 12) only received control diet without pharmacological drug.Fsurvival curve of treated mice.GImmunostaining of CD68 + LYVE-1+ macrophages (Yellow) in the aorta of surviving Ki20227-treatedJak2WT(blue) andJak2V617FMyel(green) mice (N= 8/group), scale bar 50 μm.HQuantification ofIl6, Tnfα, Il1β and Ccl2mRNA expression by RT-qPCR in the aorta of surviving Ki20227-treatedJak2WT(blue)(N=8) andJak2V617FMyel(green) (N= 7) mice.IQuantitative analysis of the mean aortic diameter of surviving Ki20227-treatedJak2WT(blue) andJak2V617FMyel(green) mice (N= 8/group) in the thoracic ascending (Asc.), thoracic descending (Desc.) and the abdominal (Abd.) aorta.JExperimental protocol describing ruxolitinib (60 mg/kg, daily during 5 weeks) or PBS treatment inJak2V617FHC-ECmice.Kquantification ofIl6, Tnfα, Il1β and Ccl2mRNA expression by RT-qPCR in the aorta ofJak2V617FHC-ECmice treated with PBS (Red) (N= 10) or Ruxolitinib (Green) (N= 8).LQuantitative analysis of the mean aortic diameter of PBS (Red,N= 7) or ruxolitinib (Green,N= 8) -treatedJak2V617FHC-ECmice using ultrasonography in the thoracic ascending (Asc.), thoracic descending (Desc.) and the abdominal (Abd.) aorta.Mexperimental protocol describing Ruxolitinib (60 mg/kg, daily during 10 weeks) or PBS treatment inJak2V617FMyelmice.Nsurvival curve of treated mice (N= 11 PBS andN= 7 Ruxolitinib). Data are presented as mean values ± SD. [Two-tailed Mann-Whitney test or Kruskal-WallisH,I, *P< 0.05, **P< 0.01, ***P< 0.001]. Difference in survival was evaluated using log-rank test. HC-EC, hematopoietic cells-endothelial cells;Il, interleukin;Tnf, tumor necrosis factor. Source data are provided as a Source Data file. Statistical analysis Values are expressed as mean ± SEM. Differences between values were examined using the nonparametric two-tailed Mann-Whitney, Kruskal-Wallis tests when appropriate and were considered significant at P < 0.05. Reporting summary Further information on research design is available in the Nature Portfolio Reporting Summary linked to this article.